The oldest known snakes from the Middle Jurassic-Lower Cretaceous provide insights on snake evolution The previous oldest known fossil snakes date from ~100 million year old sediments (Upper Cretaceous) and are both morphologically and phylogenetically diverse, indicating that snakes underwent a much earlier origin and adaptive radiation. We report here on snake fossils that extend the record backwards in time by an additional ~70 million years (Middle Jurassic-Lower Cretaceous). These ancient snakes share features with fossil and modern snakes (for example, recurved teeth with labial and lingual carinae, long toothed suborbital ramus of maxillae) and with lizards (for example, pronounced subdental shelf/gutter). The paleobiogeography of these early snakes is diverse and complex, suggesting that snakes had undergone habitat differentiation and geographic radiation by the mid-Jurassic. Phylogenetic analysis of squamates recovers these early snakes in a basal polytomy with other fossil and modern snakes, where Najash rionegrina is sister to this clade. Ingroup analysis finds them in a basal position to all other snakes including Najash . The previous understanding of the fossil record of early snake evolution (Late Mesozoic) relies on isolated vertebrae from Africa [1] (100 Myr ago), isolated jaws and vertebrae from North America [2] , [3] (98–65 Myr ago), a number of nearly complete snakes, some with rear limbs [4] , [5] , [6] , [7] , from the circum-Mediterranean region (98–95 Myr ago), and two taxa of relatively complete snakes, one with rear limbs, from Argentina (94–92 Myr ago [8] , [9] and 86–80 Myr ago [10] , [11] ). This morphologically, ecologically and phylogenetically diverse assemblage of snakes appears in the fossil record around the world almost simultaneously (~100–94 Myr ago). The long standing questions in snake palaeontology have centred on when, where and how snakes evolved and radiated from within Squamata before the early part of the Late Cretaceous. Here we report on four new species of significantly older fossil snakes (167–143 Myr ago) recognized from cranial and postcranial remains found in the United Kingdom, Portugal and the United States. These new data extend the known geological range of snakes by nearly 70 million years into the mid-Mesozoic, indicating that their origin was coincident with the known radiation of most other major groups of squamates in the mid-Jurassic [12] , [13] during the final stages of the break-up of Pangaea into Laurasia and Gondwana. It is also important to note that this new record for early snakes, co-occurring with early anguimorphs such as Dorsetisaurus [12] , [13] , fills a major chronological gap predicted by molecular phylogenetics [14] . In stratigraphic order, the oldest snake recognized here is found in rocks dated as Bathonian (~167 Myr ago), Middle Jurassic, from Southern England [15] , followed by a North American record dated as Kimmeridgian (~155 Myr ago, Upper Jurassic, Colorado, USA) [16] , which appears to be a contemporary of another taxon from the Kimmerdigian (Upper Jurassic, Guimarota, Portugal) [17] . The youngest snake taxon and materials recognized here are found in rocks dated as Tithonian (~150 Myr ago; Upper Jurassic) to Berriasian (~140 Myr ago; Lower Cretaceous) outcropping near Swanage, Dorset, Southern England [15] . Systematic palaeontology Order Squamata Opell, 1811 Suborder Serpentes Linnaeus, 1758 Parviraptor estesi gen. et sp. ( Figs 1a and 2a ; Supplementary Figs 1 and 2a–e ). 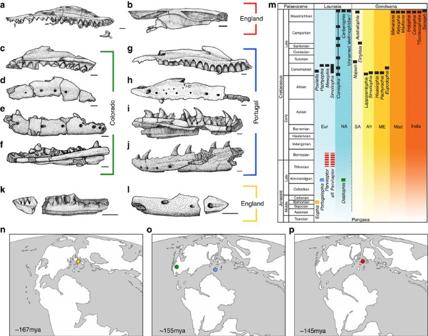Figure 1: Skull elements assigned to new genera and species of Middle Jurassic to Lower Cretaceous snakes. (a)Parviraptor estesi(NHMUK R48388, generic type), medial view left maxilla. (b) aff.Parviraptor estesi(NHMUK R8551) lateral view right frontal. (c–f)Diablophis gilmorei(c,d) medial and lateral views right maxilla (LACM 140572). (e,f) Lateral and medial views of right dentary (LACM 140572). (g–j)Portugalophis lignites(g,h) medial and lateral view left maxilla (MG-LNG 28091). (i,j) medial and lateral view left dentary (MG-LNG 28094). (k,l)Eophis underwoodi, medial and lateral views holotype (NHMUK R12355) anterior symphyseal section; paratype (NHMUK R12354) mid-dentary portion. (m) Stratigraphic and palaeobiogeographic distributions. (n) Plate tectonic reconstruction for Bathonian (~167 Myr ago), yellow dot indicates locality ofEophis underwoodi.(o) Plate tectonic reconstruction for Kimmerdigian (~155Myr ago), blue dot indicates locality ofPortugalophis lignites, green dot indicates locality ofDiablophis gilmorei.(p) Plate tectonic reconstruction for Tithonian-Berriasian (~145 Myr ago), red dot indicates locality ofParviraptor estesiand aff.Parviraptor estesi. (note: color of dots on map correspond with bracket color for specimens (a–l). Afr, Africa; Eur, Europe; Mad, Madagascar; ME, Middle East; NA, North America; SA, South America (all scale bars,a–l, 1mm). Figure 1: Skull elements assigned to new genera and species of Middle Jurassic to Lower Cretaceous snakes. ( a ) Parviraptor estesi (NHMUK R48388, generic type), medial view left maxilla. ( b ) aff. Parviraptor estesi (NHMUK R8551) lateral view right frontal. ( c – f ) Diablophis gilmorei ( c , d ) medial and lateral views right maxilla (LACM 140572). ( e , f ) Lateral and medial views of right dentary (LACM 140572). ( g – j ) Portugalophis lignites ( g , h ) medial and lateral view left maxilla (MG-LNG 28091). ( i,j ) medial and lateral view left dentary (MG-LNG 28094). ( k , l ) Eophis underwoodi , medial and lateral views holotype (NHMUK R12355) anterior symphyseal section; paratype (NHMUK R12354) mid-dentary portion. ( m ) Stratigraphic and palaeobiogeographic distributions. ( n ) Plate tectonic reconstruction for Bathonian (~167 Myr ago), yellow dot indicates locality of Eophis underwoodi. ( o ) Plate tectonic reconstruction for Kimmerdigian (~155Myr ago), blue dot indicates locality of Portugalophis lignites , green dot indicates locality of Diablophis gilmorei. ( p ) Plate tectonic reconstruction for Tithonian-Berriasian (~145 Myr ago), red dot indicates locality of Parviraptor estesi and aff. Parviraptor estesi . (note: color of dots on map correspond with bracket color for specimens ( a – l ). Afr, Africa; Eur, Europe; Mad, Madagascar; ME, Middle East; NA, North America; SA, South America (all scale bars, a – l , 1mm). 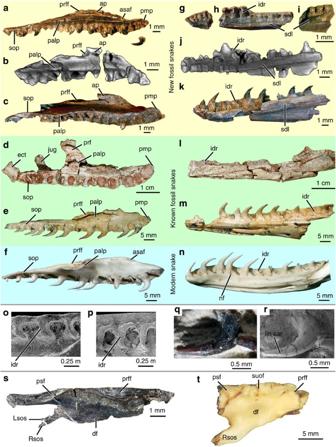Figure 2: Jaw elements of earliest snakes. (a–c,g–k) compared withDinilysia patagonica(d,l),Yurlunggursp. (e,m), and modernPythonsp. (f,n). (a) Left maxilla,Parviraptor estesi(NHMUK 48388, part). (b) Right maxilla (image reversed),Diablophis gilmorei(LACM 4684/140572, part). (c) Left maxilla,Portugalophis lignites(MG-LNEG 28091). (d) Left maxilla, prefrontal, jugal, and ectopterygoid,D. patagonica(MACN-RN 1013, part). (e) Right maxilla (image reversed),Yurlunggursp. (QMF45391, part). (f) Left maxilla,Pythonsp. (UALVP unnumbered specimen). (g)Eophis underwoodi(Holotype, R12355), anterior symphyseal section. (h)E. underwoodi(Paratype NHMUK R12354: mid-dentary portion). (i)E. underwoodi(referred specimen, NHMUK R12354: posterior dentary portion). (j) Right dentary (image reversed),D. gilmorei(LACM 4684/140572, part), new genus. (k) Left dentary (image reversed),Portugalophis lignites(MG-LNEG 28091), new gen. and sp. (l) Right dentary, splenial, angular, compound, and coronoid,D. patagonica(MACN-RN 1013, part). (m) Right dentary ofYurlunggursp. (QMF45391, part). (n) Right dentary,Pythonsp. (UALVP unnumbered specimen). (o) SEM image, posterior tooth sockets, right dentary,E. underwoodi(NHMUK R12370). (p) SEM image, posterior tooth sockets, left maxilla,Xenopeltis unicolor(FMNH 287277). (q) Light photograph, isolated left maxillary tooth with lingual apical carina,Parviraptor estesi(NHMUK 48388, part). (r) SEM image, isolated left maxillary tooth with lingual apical carina,Parviraptor estesi(NHMUK 48388, part). (s) right frontal, lateral view, aff.Parviraptor estesi(NHMUK R8551). (t) Right frontal,Pythonsp. (UALVP unnumbered specimen). ap, ascending process; asaf, anterior superior alveolar foramen; ect, ectopterygoid; idr, interdental ridges; jug, jugal; lin car, lingual carina; Lsos, left suboptic shelf; nf, nutrient foramina; palp, palatine process; pmp, premaxillary process; prf, prefrontal; prff, prefrontal facet; psf, postfrontal facet; Rsos, right suboptic shelf of frontal; sdl, subdental lamina; sop, suborbital process of maxilla; suof, supraorbital facet. Full size image Figure 2: Jaw elements of earliest snakes. ( a – c , g – k ) compared with Dinilysia patagonica ( d , l ), Yurlunggur sp. ( e , m ), and modern Python sp. ( f , n ). ( a ) Left maxilla, Parviraptor estesi (NHMUK 48388, part). ( b ) Right maxilla (image reversed), Diablophis gilmorei (LACM 4684/140572, part). ( c ) Left maxilla, Portugalophis lignites (MG-LNEG 28091). ( d ) Left maxilla, prefrontal, jugal, and ectopterygoid, D. patagonica (MACN-RN 1013, part). ( e ) Right maxilla (image reversed), Yurlunggur sp. (QMF45391, part). ( f ) Left maxilla, Python sp. (UALVP unnumbered specimen). ( g ) Eophis underwoodi (Holotype, R12355), anterior symphyseal section. ( h ) E. underwoodi (Paratype NHMUK R12354: mid-dentary portion). ( i ) E. underwoodi (referred specimen, NHMUK R12354: posterior dentary portion). ( j ) Right dentary (image reversed), D. gilmorei (LACM 4684/140572, part), new genus. ( k ) Left dentary (image reversed), Portugalophis lignites (MG-LNEG 28091), new gen. and sp. ( l ) Right dentary, splenial, angular, compound, and coronoid, D. patagonica (MACN-RN 1013, part). ( m ) Right dentary of Yurlunggur sp. (QMF45391, part). ( n ) Right dentary, Python sp. (UALVP unnumbered specimen). ( o ) SEM image, posterior tooth sockets, right dentary, E. underwoodi (NHMUK R12370). ( p ) SEM image, posterior tooth sockets, left maxilla, Xenopeltis unicolor (FMNH 287277). ( q ) Light photograph, isolated left maxillary tooth with lingual apical carina, Parviraptor estesi (NHMUK 48388, part). ( r ) SEM image, isolated left maxillary tooth with lingual apical carina, Parviraptor estesi (NHMUK 48388, part). ( s ) right frontal, lateral view, aff. Parviraptor estesi (NHMUK R8551). ( t ) Right frontal, Python sp. (UALVP unnumbered specimen). ap, ascending process; asaf, anterior superior alveolar foramen; ect, ectopterygoid; idr, interdental ridges; jug, jugal; lin car, lingual carina; Lsos, left suboptic shelf; nf, nutrient foramina; palp, palatine process; pmp, premaxillary process; prf, prefrontal; prff, prefrontal facet; psf, postfrontal facet; Rsos, right suboptic shelf of frontal; sdl, subdental lamina; sop, suborbital process of maxilla; suof, supraorbital facet. Full size image Holotype . Left maxilla on block NHMUK R48388, Natural History Museum, London. Locality horizon and age. Durlston Bay, Swanage, Dorset, England; Purbeck Limestone Formation (Upper Jurassic; Tithonian/Lower Cretaceous; Berriasian). Emended Diagnosis . Long low, ascending process of maxilla; premaxillary process turned medially; narrow prefrontal facet on ascending process of maxilla. Differs from maxilla of Coniophis precedens in lacking medial process at anterior end, in having greater degree of recurvature of teeth. Differs from Dinilysia patagonica in having gracile maxilla, relatively smaller teeth, less pronounced medial deviation at anterior tip and relatively smaller palatine process. Differs from Portugalophis lignites in having narrower premaxillary process. Differs from Diablophis gilmorei in having larger palatine process and in lacking medial curvature of anterior end of maxilla. Revised Description . Maxilla exposed in medial and dorsal views; long, 24 tooth positions preserved, bearing low ascending process extending from tooth position 4 to tooth position 16/17; anterior superior alveolar foramen large, positioned at front of ascending process; prominent premaxillary process, narrow and turned medially; supradental shelf narrow and thin with prominent palatine process adjacent to posterior end of ascending process; margin of palatine process damaged; long, tooth-bearing suborbital ramus with 10 tooth positions posterior to prefrontal facet and palatine process; maxillary tooth positions defined by three-sided alveolus with no medial border; preserved teeth attached to rims of alveoli; presence of tooth in alveolus closes small posterolingual notch forming basal nutrient foramen; teeth conical, circular cross sections, recurved, with labial and lingual carinae. aff. Parviraptor estesi ( Figs 1b , 2s and 3a ; Supplementary Figs 3a–d and 4a–i ). 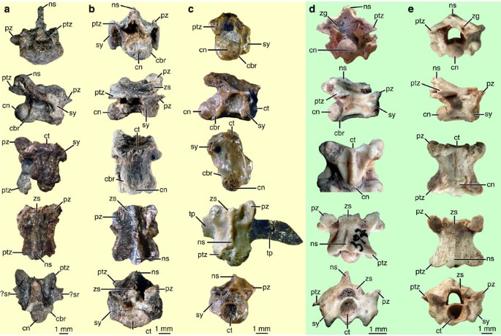Figure 3: Vertebral comparisons of earliest snakes (yellow background) toNajashandConiophis(green background) vertebrae. (a) aff.Parviraptor estesi(NHMUK R8551) in posterior, right lateral, ventral and dorsal views (note: no anterior view is available for aff.Parviraptor estesi). (b–e) Images in posterior, lateral (left forNajash, right forDiablophisandConiophis), ventral, dorsal and anterior views. (b)Diablophis gilmorei(LACM 4684/140572 [part]). (c)Diablophis gilmorei(LACM 4684/120472 [part]). (d)Najash rionegrina(MPCV 395 (ventral view), 397 (anterior, lateral [reversed for comparative purposes], dorsal views), 386 (posterior view)). (e)Coniophis precedens(UALVP unnumbered specimen). cbr, centrum bony ridge; cn, condyle; ct, cotyle; ns, neural spine; ptz, postzygapophysis; pz, prezygapophysis;?sr, possible sacral rib; sy, synapophysis; zg, zygantrum; tr, transverse process; zs, zygosphene. Figure 3: Vertebral comparisons of earliest snakes (yellow background) to Najash and Coniophis (green background) vertebrae. ( a ) aff. Parviraptor estesi (NHMUK R8551) in posterior, right lateral, ventral and dorsal views (note: no anterior view is available for aff. Parviraptor estesi ). ( b – e ) Images in posterior, lateral (left for Najash , right for Diablophis and Coniophis ), ventral, dorsal and anterior views. ( b ) Diablophis gilmorei (LACM 4684/140572 [part]). ( c ) Diablophis gilmorei (LACM 4684/120472 [part]). ( d ) Najash rionegrina (MPCV 395 (ventral view), 397 (anterior, lateral [reversed for comparative purposes], dorsal views), 386 (posterior view)). ( e ) Coniophis precedens (UALVP unnumbered specimen). cbr, centrum bony ridge; cn, condyle; ct, cotyle; ns, neural spine; ptz, postzygapophysis; pz, prezygapophysis;?sr, possible sacral rib; sy, synapophysis; zg, zygantrum; tr, transverse process; zs, zygosphene. Full size image Referred Material . Right frontal, atlas and associated precloacal vertebrae on multispecimen block NHMUK R8551 (specimen originally assigned to Parviraptor estesi [15] ). Locality, horizon and age . Swanage, Dorset, England; Purbeck Limestone Formation (Upper Jurassic; Tithonian/Lower Cretaceous; Berriasian). Description . Right frontal (NHMUK R8551) in lateral view with well-developed prefrontal and postfrontal facets and deep, medially curved descensus frontalis with well-developed suboptic shelves on posteroventral margin forming posterior portion of optic nerve foramen (Cranial Nerve II); closely associated vertebrae with tall neural spines, massive, vertical synapophyses with distinct, posteriorly expanded parapophyseal and diapophyseal facets; complete neural arch with short zygosphenes; posterior margin lacks incised median notch; elevated, round condyles with weakly constricted necks; centrum narrow posteriorly and wide anteriorly in ventral view; inferior margin of centrum, no development of haemal keel; possible sacral vertebra with robust transverse processes; left neural arch from an atlas with narrow, posteriorly directed neural spine; no notochordal canal. Remarks . Because of the loss of the provenance of this block with respect to the block NHMUK 48388, the lack of articulation of the elements, and the polytaxonomic composition of the Purbeck blocks, we do not feel that there is sufficient evidence to support referral of the frontal to type maxilla of Parviraptor estesi , although we do recognize that such a referral is a strong possibility. Diablophis gilmorei gen. nov., new combination ( Figs 1c–f and 2b,j ; Supplementary Figs 10a–k and 11a–n ; Supplementary Videos 1–9 ). Etymology . ‘ Diablo ’, ‘devil’ (Spanish); ophis , snake (Greek); in recognition of type locality near Devil’s Canyon, Colorado. Holotype . LACM 4684/140572 (Los Angeles County Museum), broken right maxilla, broken right mandible, and broken axis vertebra (revised holotype). Referred Specimens . Several precloacal vertebrae and one possible sacral vertebra LACM 4684/140572; broken right dentary LACM 5572/120732 (all specimens originally referred to Parviraptor gilmorei [16] ); LACM 4684/120472, four precloacal vertebrae, one caudal vertebra with large transverse processes. Locality, horizon and age . From Fruita locality, Morrison Formation, Mesa County, Colorado, USA (Upper Jurassic; Kimmeridgian). Diagnosis . Small-bodied snake that differs from Parviraptor estesi and Portugalophis lignites in having smaller palatine process and having strong medial deviation of anterior end of maxilla. Differs from P. lignites and from Eophis underwoodi in having more fully developed subdental lamina relative to dentary size. Differs from Coniophis precedens in the absence of medial process on anterior tip of maxilla; greater degree of recurvature of teeth; alveoli primarily on lateral parapet of dentary and maxilla; presence of subdental lamina and multiple mental foramina on dentary; and in having tall neural spines and small zygosphenes and zygantra. Description . Right maxilla (LACM 4684/140572) small, preserves 10–11 tooth spaces with broken crowns; ascending process low and long with small notch in posterior margin of apex; supradental shelf broken, thin anteriorly and thickened posteriorly; lateral surface smooth with four nutrient foramina; alveoli/interdental ridges with incised medial walls forming nutrient notch; tooth crowns conical, recurved, sharp; holotype right dentary missing symphysis and postdentary articulation region; straight in dorsal view with medial turn anteriorly and 11 tooth spaces; well-developed subdental lamina forming medial border of subdental gutter; lateral wall with seven mental foramina; dentary teeth attached to three-sided alveoli; teeth circular in cross-section, conical and strongly recurved; neural spine tall, synapophyses massive and vertical, and condyle elevated above bottom of centrum; neural canals show ‘trefoil’ organization often present in snakes [3] , [8] ; condyle round, with weakly constricted neck and synapophysis with posteriorly expanded parapophyseal and diapophyseal facets; centrum narrow posteriorly, wide anteriorly; inferior margin of centrum without haemal keel; paralymphatic fossae present; no notochordal canal; small zygosphene-zygantrum articulations. Eophis underwoodi gen. et sp. nov. ( Figs 1k,l and 2g–i ; Supplementary Figs 5a–i and 6a–g ). Etymology. Eos , dawn (Greek); ophis , snake (Greek); underwoodi (Surname); in recognition of being oldest known snake material, and lifelong impact/contributions of Garth Underwood to study of snakes. Syntypes . NHMUK R12355, symphyseal portion of right dentary; NHMUK R12354, midsection right dentary; NHMUK R12370, posterior portion right dentary (all three specimens previously referred to Parviraptor cf. P. estesi [15] ). Referred specimen. NHMUK R12352, fragment of left maxilla. Locality, horizon and age . Forest Marble, Kirtlington Cement Works Quarry, Oxfordshire, England (Middle Jurassic; Bathonian). Diagnosis . Small-bodied snake with low and shallow subdental lamina of dentary. Differs from both Diablophis gilmorei and Portugalophis lignites in having smaller subdental lamina relative to dentary size. Differs from Coniophis precedens in having a subdental lamina, and multiple mental foramina on dentary. Description . Dentary fragments with three-sided alveoli forming distinct interdental ridges and tall lateral parapet; medial side of alveolus with nutrient notch; short subdental lamina and well-developed Meckelian fossa, narrow anteriorly, wide posteriorly; intramandibular septum fused to floor of Meckelian fossa; mandibular symphysis smooth and broad; lateral surface of dentary convex with 4 – 5 mental foramina; NHMUK R12370 possesses narrow facet on medial edge of subdental lamina for articulation with anteromedial process of coronoid; ventromedial edge of dentary with narrow facet for articulation with splenial. NHMUK R12352 ( Supplementary Fig. 6e–g ) is a fragment of the left maxilla preserving three alveoli and an incomplete portion of the dorsal process. The most complete alveolus is similar to those of the dentary in being three-sided with the interdental ridge canal (irc) piercing the alveolar bone between adjacent alveoli. A small tooth is lodged within the irc. Portugalophis lignites gen. et sp. nov. ( Figs 1g–j and 2c,k ; Supplementary Figs 7a–j,8a–c and 9a–c ; Supplementary Videos 10–14 ). Etymology . Portugal , Portugal; ophis , snake (Greek); lignites , lignum (Latin); in recognition of Portugal, snake affinities, and coal-lithology of Guimarota Mine. Holotype . Left maxilla (holotype), MG-LNEG 28091 (Museu Geologico, Lisboa, Portugal). Paratype. MG-LNEG 28094, left dentary. Referred Specimen. MG-LNEG 28100, partial left maxilla. Locality . From coal beds, Guimarota mine, Leiria, Portugal (Upper Jurassic; Kimmeridgian). Diagnosis . Differs from Parviraptor estesi, Eophis underwoodi , and Diablophis gilmorei in larger size, dentary tooth bases extend into subdental gutter. Further differs from P. estesi in having wider premaxillary process of maxilla, more deeply concave medial surface of ascending process of maxilla. Differs from Eophis underwoodi in having taller subdental lamina relative to dentary size. Differs from Coniophis in the absence of medial process on anterior tip of maxilla; greater degree of recurvature of teeth; alveoli primarily on lateral parapet of dentary and maxilla; and the presence of subdental lamina and multiple mental foramina on dentary. Description. MG-LNEG 28091, holotype left maxilla, ascending process long and low with dorsal edge turned medially; ascending process with distinct, broad facet and notch for prefrontal; maxilla with two rows of labial foramina, inferior row large, superior row small; premaxillary process short, broad, mediolaterally expanded with opening of anterior superior alveolar foramen at posterior margin; supradental shelf narrow and rounded with distinct medially expanded palatine process (between tooth positions 11 and 15); 15 preserved alveoli with 9 fragmentary teeth; alveoli with tall lateral walls, well-defined three-sided alveolar margins and interdental ridges, and low medial wall notched by nutrient foramen; paratype dentary, MG-LNEG 28094, with 15 tooth spaces and 6 teeth; well-developed subdental lamina thickened posteriorly bordering large and prominent sulcus dentalis; posteriorly, subdental lamina with narrow splenial facet; Meckelian fossa tall posteriorly, narrowing to form shallow channel, open ventrally; anteriormost portion of lateral emargination preserved; 5–6 large, circular mental foramina; teeth conical, sharply pointed, strongly recurved, and bear anteromedial and posterolateral carinae; tooth bases broad, set in margins of tooth sockets/alveoli. Comparative anatomy of early snakes These new snake taxa are based on specimens that were either previously described and named, or referred to, various species or groups of anguimorph lizards [15] , [16] , [17] . The problems associated with identifying any of the Parviraptor specimens as the remains of snakes were due to the fact that the original taxon [15] was a complex chimaera (see Supplementary Figs 12–23 ; Supplementary Notes 1,2 ). The type species, P. estesi [15] was assembled from isolated to arguably associated fossils preserved on two different blocks of rock, NHMUK R48388 from slightly older strata at Durlston Bay, Swanage, the United Kingdom [15] ( Supplementary Fig. 1 ) and NHMUK R8551 from younger strata at Swanage, the United Kingdom [15] ( Supplementary Fig. 3 ). The original characterization of Parviraptor cf. P. estesi [15] was based on isolated specimens found more than 150 km away at Kirtlington, Oxfordshire, the United Kingdom ( Fig. 1n ), in rocks that are ~30 million years older than the type and referred block ( Fig. 1p ). Reinterpretation of these specimens finds that the original type and referred specimens of Parviraptor estesi [15] and Parviraptor cf. P. estesi [15] include the remains of possibly three separate taxa of snakes, a large number of gekkotan as well as other indeterminate lizard elements, and also a number of non-squamate elements and one invertebrate fragment ( Supplementary Figs 12–23 ). The identity and affinities of Parviraptor were further confounded by recent phylogenetic investigations that, based on the original descriptions [15] , found the taxon to have gekkotan affinities [18] , [19] . These hypotheses arose from the assignment to Parviraptor cf. P. estesi [15] of gekkotan vertebrae from the Kirtlington Quarry ( Supplementary Figs 20–23 ) that bear notochordal canals piercing the centra, as well as amphicoelous condyles/cotyles; it is important to note that no such vertebrae occur on either the original Swanage type block, NHMUK R8551, or the referred block NHMUK R48388. In addition, the isolated parietals preserved on the Swanage blocks ( Supplementary Fig. 13 ) are identified here as gekkotan, which explains the character scorings for Parviraptor as a gekkotan [18] , [19] , in contrast to the original description [15] . The original descriptions of Diablophis gilmorei [16] and Portugalophis lignites [17] avoided the chimaera problem of Parviraptor estesi /aff. Parviraptor [15] as the materials selected from the microvertebrate assemblages were only compared with the maxilla and teeth of P. estesi . Identifying the affinities of disarticulated vertebrate remains is difficult and relies on detailed comparisons of specialized features that characterize one vertebrate over another. However, snakes possess a number of detailed cranial and postcranial anatomies that are definitively characteristic of the group, distinguishing them from other squamates, and that are present in these new Middle Jurassic–Lower Cretaceous forms. The unique features of snake cranial, dental and axial skeletal elements make it possible to identify snakes in the fossil record from isolated or even fragmentary elements [2] , [3] , [20] . Skull, jaw and dental features characterizing fossil and modern snakes [21] that are present in the oldest snakes described here ( Figs 1a–l and 2a–t ; Table 1 ; Supplementary Figs 1–11 ; Supplementary Videos 1–6 and 11–14 ), recognizing of course the limits imposed by incompleteness and preservation, include (1) long, tooth-bearing sub-orbital ramus of maxilla, unique to snakes with exception of some gekkos ( Fig. 2a,c–f ; Supplementary Figs 2a–c and 7a–f ; Supplementary Videos 1, 2, 10–12 ); (2) distinct and medially projecting palatine process of maxilla lacking supradental shelf as present in lizards ( Fig. 2a–f ; Supplementary Fig. 2a–c ; Supplementary Videos 1, 2, 10–12 ); (3) prefrontal facets on ascending process of maxilla anterior to palatine process ( Fig. 2a–f ; Supplementary Video 1, 2, 10–12 ); (4) low and rounded ascending process of maxilla, with small medial facets for prefrontal ( Fig. 2a–f ; Supplementary Figs 2a–c and 7a–f ; Supplementary Video 1, 2, 10–12 ); (5) lateral dentary wall emarginated, resulting in exposure of anterior (‘prearticular’) portion of compound bone ( Supplementary Figs 7g and 8c ; Supplementary Videos 13, 14 ); (6) dorsal position and superior exposure of anterior opening of superior alveolar canal (anterior superior alveolar foramen) along anterodorsal margin of maxilla (in lizards, this feature is variably projecting medially, and is covered by nasals, septomaxilla, or overhanging ascending process of maxilla) ( Fig. 2a–f ; Supplementary Figs 7e and 9a ); (7) smooth and rounded anteromedial process of maxilla for ligamentous connection with premaxilla ( Fig. 2a–f ; Supplementary Videos 10–12 ); (8) well-developed descensus frontalis and posteriorly, suboptic shelves ( Fig. 2s–t ; Supplementary Fig. 3c,d ); (9) strongly recurved maxillary and dentary teeth where maxillary teeth are more recurved than the dentary teeth; a sigmoidal curvature cannot be observed; however, such curvature is not present in all snakes and can also disappear ontogenetically (see for example, Fig. 2a,c,k with Fig. 2e,f,m,n ; Supplementary Figs 2a–c and 8c ; Supplementary Videos 1–4 and 10–12 ); (10) short tooth root, with enamel cap not extending to cementum margin; (11) small posterolingual nutrient foramen at margin of alveolus (in lizards, nutrient foramina, when present, are bounded, at least partially, by base of tooth); (12) alveoli three-sided, alveolar bone forming interdental ridges and lining lateral parapet ( Figs 1a–l and 2a–p ; Supplementary Fig. 6a–d ; Supplementary Videos 1–4 and 10–12 ); (13) labial and lingual carinae on apex of tooth crowns ( Fig. 2a,k,e–n,q,r ; Supplementary Fig. 2b,d,e ). Table 1 Distribution in new fossil taxa of diagnostic cranial features present in some or all modern and fossil snakes. Full size table Comparison of the alveolar walls of Eophis underwoodi with those of the modern snake Xenopeltis unicolor ( Fig. 2o,p ; Supplementary Fig. 6a–d ) shows a striking similarity in the construction between the two taxa. In both taxa the interdental ridge is continuous posteriorly with the lateral parapet to form a J-shaped boundary to the alveolus. An obvious difference between the jaws of the oldest known snakes and geologically younger snakes is the presence of a maxillary supradental shelf ( Fig. 2a–c ) and distinct dentary subdental shelf and sulcus dentalis that runs the length of the tooth-bearing element ( Fig. 2g–k ). In modern snakes, inclusive of scolecophidians, and geologically younger snakes such as Yurlunggur , the medial bony tissues of the maxilla and dentary grade smoothly [20] , [21] into the tooth row without forming a shelf ( Fig. 2d–f,l–m ) though a small shelf persists on the dentary immediately superior to the articulation with the posterior portion of the splenials ( Fig. 2l–m ). Fossil snakes such as Dinilysia are similar to the oldest known snakes, while Coniophis is more similar to Yurlunggur . Associated with the tooth bearing elements of Diablophis gilmorei , is a small elongate element that appears to be the right surangular bone ( Supplementary Fig. 10i–k ); the element was not included in the parsimony analysis as the association is weak. However, this disarticulated surangular is long, bears a large snake-like adductor fossa and laterally directed coronoid process, but is not fused into a single compound bone (thus, the articular surface for the quadrate is only partly preserved, as the articular bone is missing). It may well be that ~140 Myr ago the compound bone characteristic of all other fossil and modern snakes [20] , [21] had not yet appeared in snake evolution. Vertebral features that are present in two of the new fossil snakes (aff. Parviraptor estesi ; Diablophis gilmorei ) and are shared with fossil snakes such as Najash rionegrina and Coniophis precedens [2] , [3] ( Fig. 3a–e ; Table 2 ; Supplementary Figs 4a–g and 11a–n ), but not necessarily with all fossil and modern snakes include (1) well-developed synapophyses continuous with prezygopophysis; (2) synapophyses divided into dorsal and ventral surfaces; (3) all four snakes lack accessory processes on the prezygapophyses, and the synapophyses are lateral, not ventral as in more modern snakes; (4) the synapophyses flare laterally from the cotylar margin, while posteriorly the centrum is expanded mediolaterally just in front of the condyle (except C. precedens ); (5) small zygosphenes and zygantra are present in both D. gilmorei and aff . Parviraptor estesi ; the zygosphene articulations are present, small, set on a narrow neural arch platform and not as well developed as they are in Coniophis and Najash ; (6) the possession of a ‘trefoil’ organization of the neural canal [3] ; (7) round condyle and cotyle; (8) constriction at base of condyle; (9) long, broad, transverse processes on postcloacal vertebrae. Table 2 Distribution in fossil taxa of diagnostic vertebral features of snakes. Full size table The features shared by aff. Parviraptor estesi and Diablophis gilmorei with Najash rionegrina and the much younger (~100 Myr difference) Coniophis precedens are interesting and important, despite the much weaker development of the zygosphene-zygantral articulations and width of neural arch platform in the first two snakes ( Fig. 3a–e ; Supplementary Figs 4a–g and 11a–n ). However, in contrast to most known snakes [8] , [9] , there is one potential sacral vertebra present on the aff. Parviraptor estesi (NHMUK R8551) slab ( Fig. 3a ) and another in the vertebral specimens referred to Diablophis gilmorei (4684/140572). Each vertebra is far more robust than the materials described for Najash rionegrina [8] , [9] ( Fig. 3d ), suggesting the possible presence of robust pelvic girdles and hind limbs. The referred postcloacal vertebra of D. gilmorei (LACM 4684/120472) possesses a large transverse process that is directed laterally, not anteriorly as in modern snakes, and is more similar in size and orientation to postcloacal transverse processes of Najash . As this report extends the fossil record of snakes by ~70 million years, it is likely that these early snakes shared with younger fossil snakes [4] , [7] , [8] the presence of at least rear limbs. However, we remain conservative on this point and have not coded this information for phylogenetic analysis ( Supplementary Information Section 3); presence or absence of forelimbs remains mere speculation as it cannot be verified by reference to current specimens. Phylogeny At the alpha taxonomic level, based on comparative anatomy, Parviraptor , Diablophis , Eophis and Portugalophis are confidently identified as snakes [1] , [2] , [3] , [20] , [22] , [23] , [24] . However, to address questions of phylogeny, we conducted two separate analyses using two vastly different data matrices. To test the possibility that these new snakes might fall outside of the snake clade in an overall analysis of squamate phylogeny, we included them in a recent large matrix of all squamates [25] . We also examined the more specific characters related to snakes, by including them in a data matrix originally developed to test snake ingroup relationships [3] , [7] , [8] , [26] , [27] , [28] ( Supplementary Methods ; Supplementary Dataset 1 ). Both phylogenetic analyses were run using the software programs PAUP [29] and TNT [30] , the latter was also used to calculate bootstrap values of statistical support. The matrix [25] analysed in our examination of overall squamate phylogeny included the addition of the maxillae of Parviraptor , Portugalophis and Diablophis as terminal taxa (the maxillae were selected because, of all the isolated elements, they are those that allow for the largest number of character states that can be coded; other elements associated with these maxillae were not included to provide the strictest test of phylogenetic relationships); the goal of this analysis was to test whether or not these partial skeletal remains would be recovered as snakes, or fall outside that clade. In the strict consensus tree of 108,981 shortest trees retrieved in PAUP [29] (tree length: 5290 steps), all three taxa were reconstructed within a polytomy comprised of Mesozoic snakes ( Dinilysia , Pachyrhachis , Haasiophis and so on), scoleocophidians and alethinophidians, with Najash as the most basal snake. The strict consensus of 200 trees retrieved using TNT [30] (tree length: 5283) is very similar to the strict consensus of the trees retrieved in PAUP [29] , and the only differences consist in the repositioning of some basal macrostomatans (for example, Calabaria , Eryx and Lichanura ) and in the addition to the basal polytomy of the taxa Casarea , Xenophidion , Loxocemus and Xenopeltis . The clade Ophidia (that is, all extant and fossil snakes) was retrieved with strong bootstrap support (BS=85) ( Fig. 4a ; Supplementary Methods ). These results are supportive of our identification of these specimens as the remains of snakes, and that derived features of snakes were present among squamates as early as the Middle to Upper Jurassic. 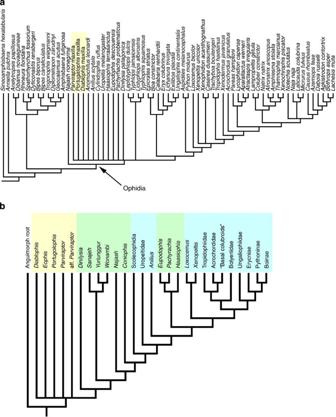Figure 4: Phylogeny of earliest known snakes and other fossil and living snakes. (a) Snake portion of Strict Consensus Tree of 108,981 shortest trees, illustrating overall phylogeny of squamates25includingParviraptor,DiablophisandPortugalophis(yellow background). All three taxa are nested within a polytomy comprised Mesozoic snakes (Dinilysia,Pachyrhachis,Haasiophisand so on), scoleocophidians and alethinophidians, withNajash9as the basal most snake. Tree length (TL)=5290; consistency index (CI)=0.1841; homoplasy index (HI)=0.8159; retention index (RI)=0.7934; Bootstrap support for clade Ophidia: 85. (b) Tree derived from Strict Consensus Tree of 305 most parsimonious trees (MPTs) retrieved by parsimony analysis of matrix composed of 27 terminal taxa of fossil and living snakes, and 237 characters (tree length (TL)=515; consistency index (CI)=0.5340; homoplasy index (HI)=0.4660; retention index (RI)=0.6935). Terminal taxon ‘Coniophis’ (vertebrae, left maxilla, right dentary only) reconstructed in sistergroup position to all extant snakes with fossil clade Pachyophiidae nested within that extant clade. The earliest snakes (yellow background) form a clade as sistergroup to all other snakes, fossil (green background) and modern (blue background), in 98 of 305 MPTs. In remaining 207 MPTs, the earliest snakes form a paraphyletic assemblage belowDinilysia. Figure 4: Phylogeny of earliest known snakes and other fossil and living snakes. ( a ) Snake portion of Strict Consensus Tree of 108,981 shortest trees, illustrating overall phylogeny of squamates [25] including Parviraptor , Diablophis and Portugalophis (yellow background). All three taxa are nested within a polytomy comprised Mesozoic snakes ( Dinilysia , Pachyrhachis , Haasiophis and so on), scoleocophidians and alethinophidians, with Najash [9] as the basal most snake. Tree length (TL)=5290; consistency index (CI)=0.1841; homoplasy index (HI)=0.8159; retention index (RI)=0.7934; Bootstrap support for clade Ophidia: 85. ( b ) Tree derived from Strict Consensus Tree of 305 most parsimonious trees (MPTs) retrieved by parsimony analysis of matrix composed of 27 terminal taxa of fossil and living snakes, and 237 characters (tree length (TL)=515; consistency index (CI)=0.5340; homoplasy index (HI)=0.4660; retention index (RI)=0.6935). Terminal taxon ‘ Coniophis ’ (vertebrae, left maxilla, right dentary only) reconstructed in sistergroup position to all extant snakes with fossil clade Pachyophiidae nested within that extant clade. The earliest snakes (yellow background) form a clade as sistergroup to all other snakes, fossil (green background) and modern (blue background), in 98 of 305 MPTs. In remaining 207 MPTs, the earliest snakes form a paraphyletic assemblage below Dinilysia . Full size image In our parsimony analyses of snake ingroup phylogeny, we submitted a taxon-character matrix of 27 terminal taxa and 237 characters, derived in large part from a recent study [3] that in turn had adapted characters and taxa from several other works [8] , [11] , [24] , [26] , [27] , [31] ( Supplementary Methods ; Supplementary Dataset 1). Our characterization of the Upper Cretaceous snake, Coniophis precedens [3] is more conservative than that given in a recent report [3] , and is restricted to the vertebral assemblage, a single maxillary fragment (the other maxillary fragments are identified here as lizards, not snakes) and a fragmentary right dentary [3] , [24] . We also followed the more restrictive concept of Najash [8] in coding that taxon as was recently suggested in a conservative revision of the materials assigned to the type of that taxon [9] (Supplementary Dataset 1). The results of our ingroup phylogenetic analysis suggest that the new Jurassic/Lower Cretaceous fossil snakes either form a clade in the sistergroup position to all other known snakes, or form a paraphyletic assemblage at the base of the radiation of all other snakes ( Fig. 4b ). The new data, and the results of our analysis of snake phylogeny (see also Supplementary Figs 24 and 25 ), agree with previous ingroup analyses of fossil snakes [3] , [4] , [8] , [26] , [27] , [28] , [31] that hypothesized that the most basal snakes are not the extant scolecophidians [7] , [32] . The new early snakes add to those hypotheses by extending the fossil record of snakes by 70 million years ( Fig. 1m–p ) coincident with the radiation of other mid-Jurassic squamate groups [12] , [13] and with molecular clock predictions [14] . Paleobiogeography An extension of the fossil record of snakes to the Middle Jurassic is not surprising, as it coincides with the radiation of other major groups of squamates [12] , [13] , even though these new records of diverse and broadly distributed mid-Mesozoic (~167–145 Myr ago) snake assemblages ( Fig. 1m–p ) create a significant temporal gap with the previous early records of snakes (~100 Myr ago) from Africa [1] , North America [2] , Brazil [32] and Europe [33] . An unexpected result is the paleoecological and paleobiogeographical diversity and distribution of these Middle Jurassic–Early Cretaceous snakes ( Fig. 1m–p ). These earliest snakes are found preserved in rocks deposited in coal swamps ( Portugalophis ) [17] , mixed coastal lake and pond systems ( Eophis, Parviraptor , aff. Parviraptor ), river systems ( Diablophis ) [16] and on epicontinental islands located up to several hundred kilometers off the coastline of the closest large landmass ( Fig. 1n–p ). Subsequent snakes appear in rocks deposited in fluvial [1] , [2] , [3] , [8] , [9] , [10] , [11] and marine environments [4] , [5] , [6] , [7] , making the paleogeography and paleoecology of the earliest snakes into important reference points for later evolutionary radiations. It is possible that these early snakes were isolated on various islands and continents during the break-up of Pangaea in the mid-Mesozoic ( Fig. 1n ). Such a scenario finds support based on the similarities of their cranial features to those of Dinilysia [10] , [11] and later madtsoiids [22] , [26] , [27] , [28] ( Fig. 2a–p ), which certainly appear to be restricted to Gondwana continents during the Mesozoic and Cenozoic. It is also possible that snakes forming these island assemblages arrived as secondarily aquatic invaders. Secondary invasions of marine environments certainly characterize the subsequent evolutionary histories of numerous clades of fossil and modern snakes [4] , [5] , [6] , [31] . In fact, there is no evidence to suggest that these radiation scenarios are mutually exclusive, and so it is possible that both Pangaean-derived vicariance and multiple adaptive radiations (marine and terrestrial) influenced the Jurassic radiation of snakes and the subsequent Gondwanan and Laurasian evolution of these animals through the Mesozoic and Cenozoic [4] , [5] , [6] , [7] , [8] , [9] , [10] , [11] . These earliest snakes provide insights on aspects of snake origins, adaptive radiations, phylogeny and evolution. A recent study on the Late Cretaceous snake Coniophis precedens concluded that the snake body evolved before the snake head [3] ; this conclusion was based on supposed lizard-like features observed in isolated and disassociated skull elements linked to similarly isolated vertebrae from numerous individuals collected at two disparate localities. Observations of living groups of lizards and snakes suggest the opposite transformation of morphology from that proposed in a recent study of material referred to Coniophis [3] , that is, that the snake skull evolved before the elongate and limb-reduced to limbless postcranial skeleton. For example, scincid lizards, whether fully limbed and short-bodied, or limb-reduced to limbless and elongate, are diagnosable as scincid lizards by their distinctive skull anatomy. This is also true for all limb-reduced to limbless anguids, cordylids, gerrhosaurids, gymnophthalmids and pygopodids [34] , [35] . Because snakes are lizards, nested within that monophyletic assemblage [31] , it is possible to extend this analogy as a test of the conclusions presented in the aforementioned Coniophis study [3] . The observation that ‘skinkness’ or ‘anguidness’ is diagnosed not by elongation and limb reduction to limblessness, but rather by the shared possession of anatomical features of the head, and the recognition that snakes are lizards, leads to the prediction that the fossil record of snake evolution will likely reveal four legged, short bodied, ‘stem-snakes’ that possess ‘snake’ skull anatomies. Such a prediction is logically consistent with the pattern seen in all groups of living limbless to limb-reduced lizards; the recent claim to the contrary [3] violates that prediction and would be extraordinary if supported by fossil evidence. While we cannot ascertain the shape, length, form and so on of any aspect of the body of the earliest snakes (~167 Myr ago) reported herein, these animals are, however, identifiable as snakes by their cranial features. If ‘snakeness’ is recognized in the numerous cranial features of the ~167–143 Myr ago snakes described herein, nearly 100 million years before Coniophis precedens [3] , and if cranial features diagnose squamate groups regardless of postcranial evolution, then the prediction given here is that evolution of the snake skull was the key innovation of the clade, and not elongation and limb reduction, contrary to previous claims [3] . By the Middle Jurassic–Lower Cretaceous, and amidst the break-up of the old supercontinent Pangaea, snakes were distinguished from their lizard relatives by the possession of a skull with snake cranial and dental features that are certainly present by the Cenomanian [4] , [5] , [6] , [7] and are retained to the present. Similar to many lineages of squamates [34] , [35] , it seems likely that they then subsequently evolved elongate and limb-reduced to limbless bodies, evolving and adapting through more than 167 million years of earth history to become the extremely diverse group they are today. Materials examined The specimens of fossil (13 taxa) and living snakes (76 taxa) examined in this study belong to the collections of the following institutions: American Museum of Natural History, New York, USA (AMNH); Field Museum of Natural History, Chicago, Illinois, USA (FMNH); Hebrew University of Jerusalem, Paleontology Collections (HUJ-PAL); Museo Argentino de Ciencias Naturales ‘Bernardino Rivadavia’, Buenos Aires, Argentina (MACN-RN); Museum of Comparative Zoology, Cambridge, Massachusetts, USA (MCZ); Museo de La Plata, La Plata, Argentina (MLP); MPCA, Museo Provincial Carlos Ameghino, Cipolletti, Río Negro, Argentina (MPCA-PV); Museo di Storia Naturale di Milano, Milano, Italy (MSNM); Natural History Museum, London, UK (NHML); Naturhistoriches Museum, Vienna, Austria (NMV); Queensland Museum, Brisbane, Australia (QMF); Natural History Museum of Gannat, Gannat, France (Rh-E.F.); Senkemberg Museum, Frankfurt, Germany (SMF); University of Alberta Zoology Museum (UAZM); University of Florida, Gainesville, Florida, USA (UF); National Museum of Natural History, Washington, DC, USA (USNM); Zoologisches Forschungsmuseum Alexander Koenig, Bonn, Germany (ZFMK). The thirteen fossil snake taxa include Eupodophis descouensi Rh-E.F. 9001, 9002, 9003, MSNM V-3660, 3661, 4014; Haasiophis terrasanctus HUJ-PAL 659; Pachyrhachis problematicus HUJ-PAL 3659, HUJ-PAL 3775; Dinilysia patagonica MLP 26-410, MPCA-PV 527; MACN-RN-976, 1013, 1014; Yurlunggur sp. QMF 45391; Najash rionegrina MCPA-PV 380-388, 389–400; Sanajeh indicus 26 ; Wonambi naracoortensis SAM 30178; Parviraptor estesi NHMUK 48388; Portugalophis lignites MG-LNEG 28091, 28094, 28100; Eophis underwoodi NHMUK R12355, R12354, R12370; Diablophis gilmorei LACM 4684/140572, 4684/140572, 5572/120732; aff. Parviraptor estesi NHMUK R8551; Pachyophis woodwardii NMV A3919. Additional anatomical features were observed by reference to CT scans available through www.digimorph.org ( Aspidoscelis tigris; Anomochilus leonardi; Cylindrophis rufus; Uropeltis woodmasoni; Anilius scytale; Xenopeltis unicolor; Loxocemus bicolor; Typhlops jamaicensis; Leptotyphlops dulcis; Python molurus; Boa constrictor; Casarea dussumieri; Ungaliophis continentalis; Lichanura trivirgata; Calabaria reinhardtii; Naja naja; Thamnophis marcianus; Natrix natrix) , and from MicroCT scans completed by the authors ( Anomalepis flavapices ; Atractaspis aterrima) . Phylogenetic analysis The sistergroup and ingroup relationships of fossil and modern snakes were approximated using parsimony methods in both PAUP and TNT. The sistergroup relationships of Parviraptor , Portugalophis and Diablophis , and a large sample of other fossil and modern snake terminal taxa, were tested using the matrix and methods (for example, ordering, outgroup selections and so on) of a recent study testing overall squamate relationships [25] . Sixteen characters were coded in that matrix [25] for the maxillary elements of the three fossil snake taxa described here (see Supplementary Methods for details). The ingroup relationships of snakes, including the fossil taxa described here, were tested using a significantly modified data matrix (see Supplementary Methods ; Supplementary Dataset 1) from a recent study reporting on the phylogenetic relationships of the Mesozoic snake taxon, Coniophis [3] . The same outgroup taxon was used as was employed in that previous study [3] , although with some modifications to the coding for the ‘anguimorph root’ [3] . Contra the previous study [3] , all characters were analysed unordered and unweighted in both matrix tests. The data were analysed using the Heuristic Search option in PAUP* 4.0b (ref. 29 ) and character transformations were optimized using the ACCTRAN assumption. The data set was also tested using two different search routines in TNT [30] ; the Traditional search and the Drift search option from the New Technology searches. The Traditional search was run using 100 Wagner seed trees, 100 replications, but no swapping algorithims were utilized (for example, SPR, TBR) as the data set is not excessively large. The Drift search was chosen because unlike the Ratchet option it does not reweight characters during the analysis. This analysis was run using the default settings for the search. Nomenclatural acts This published work and the nomenclatural acts it contains have been registered in ZooBank, the proposed online registration system for the International Code of Zoological Nomenclature (ICZN). The ZooBank LSIDs (Life Science Identifiers) can be resolved and the associated information viewed through any standard web browser by appending the LSID to the prefix ‘ http://zoobank.org/ ’. The LSIDs for this publication are: urn:lsid:zoobank.org:act:FDF73A76-1B5C-43C4-957B-479568D7B478; urn:lsid:zoobank.org:act:5513C88B-AB09-4929-8501-5341EA3DDF46; urn:lsid:zoobank.org:act:8B66D02D-CC1A-4DAA-B927-7C5D450272C6; urn:lsid:zoobank.org:act:A5F66167-1EF0-4FAE-8723-DF5912D7CF18. How to cite this article : Caldwell, M. W. et al . The oldest known snakes from the Middle Jurassic-Lower Cretaceous provide insights on snake evolution. Nat. Commun. 6:5996 doi: 10.1038/ncomms6996 (2015).